The insulin and IGF1 receptor kinase domains are functional dimers in the activated state The insulin receptor (IR) and insulin-like growth factor-1 receptor (IGF1R) are highly related receptor tyrosine kinases with a disulfide-linked homodimeric architecture. Ligand binding to the receptor ectodomain triggers tyrosine autophosphorylation of the cytoplasmic domains, which stimulates catalytic activity and creates recruitment sites for downstream signalling proteins. Whether the two phosphorylated tyrosine kinase domains within the receptor dimer function independently or cooperatively to phosphorylate protein substrates is not known. Here we provide crystallographic, biophysical and biochemical evidence demonstrating that the phosphorylated kinase domains of IR and IGF1R form a specific dimeric arrangement involving an exchange of the juxtamembrane region proximal to the kinase domain. In this dimer, the active position of α-helix C in the kinase N lobe is stabilized, which promotes downstream substrate phosphorylation. These studies afford a novel strategy for the design of small-molecule IR agonists as potential therapeutic agents for type 2 diabetes. The insulin receptor (IR) and insulin-like growth factor-1 receptor (IGF1R) are members of the receptor tyrosine kinase (RTK) family of cell-surface receptors [1] and play critical roles in metabolism and cell growth [2] , [3] . Unlike canonical RTKs, these receptors are disulfide-linked homodimers in which each protomer consists of an extracellular α subunit and a membrane-spanning β subunit, which contains the cytoplasmic tyrosine kinase domain. Insulin or IGF1 binding to the extracellular region (ectodomain) of its cognate receptor triggers the autophosphorylation (in trans ) of tyrosine residues in the cytoplasmic domains [4] , which increases the catalytic (phosphoryl transfer) activity of the receptor and creates phosphotyrosine recruitment sites for downstream signalling proteins such as the IR substrate (IRS) proteins [5] . The mechanisms by which ligand binding to the ectodomains of IR and IGF1R facilitate the autophosphorylation of the cytoplasmic domains are not well understood. A structure of the dimeric IR ectodomain in the insulin-free (basal) state has been determined [6] , as well as a structure of insulin bound to its primary site on a truncated IR ectodomain [7] . These structures, although highly informative, do not fully reveal the conformational changes induced by insulin. Two recent studies offer conflicting models for the insulin-induced conformational change in the receptor. In one study [8] , experiments with a peptide representing the transmembrane helix of IR suggested that the transmembrane helices are dimerized in the basal state, and that insulin binding induces a conformational change that separates them. In the other study [9] , based on fluorescence resonance energy transfer (FRET) and cysteine-crosslinking data for IGF1R, the opposite behaviour of the transmembrane helices was proposed: dimerization on ligand binding. In either case, it is not known how the two cytoplasmic kinase domains are disposed in the basal state such that trans -phosphorylation is limited. Also unresolved is whether, on insulin-induced autophosphorylation, the two phosphorylated kinase domains function independently or in tandem to phosphorylate downstream substrates. Several crystal structures of the IR and IGF1R kinase domains have been determined in their unphosphorylated [10] , [11] (low activity) and phosphorylated [12] , [13] (activated) forms. These structures, along with biochemical studies, have illuminated two mechanisms of cytoplasmic-domain autoinhibition: the major one involving the kinase activation loop [12] , and a second one involving the juxtamembrane region [14] , [15] , which links the kinase domain to the transmembrane helix. Both autoinhibitory mechanisms are relieved through trans -phosphorylation of the activation loop [4] . Here we present a crystal structure of the IR kinase domain and the preceding juxtamembrane region in a phosphorylated state. The presence of a symmetric dimer in the structure, in which the juxtamembrane region of one molecule interacts with an important regulatory element, α-helix C, in the kinase domain of the other molecule, suggests the possibility that the phosphorylated kinase domains of IR and IGF1R function as dimeric units for optimal substrate phosphorylation. We verified this hypothesis through in vitro biochemical and biophysical studies and through in-cell functional assays. Thus, we show that the kinase domains of IR and IGF1R are regulated allosterically through dimer formation as well as by tyrosine phosphorylation of the activation loop. Crystal structure of IR-JMTK We determined a crystal structure at 2.3-Å resolution of the juxtamembrane region and tyrosine kinase domain of IR (referred to as IR-JMTK), residues 956–1283 (numbering for isoform IR-B), in which Tyr972 in the juxtamembrane region (recruitment site for IRS proteins) and Tyr1158, Tyr1162 and Tyr1163 in the activation loop of the kinase domain were phosphorylated in vitro before crystallization. 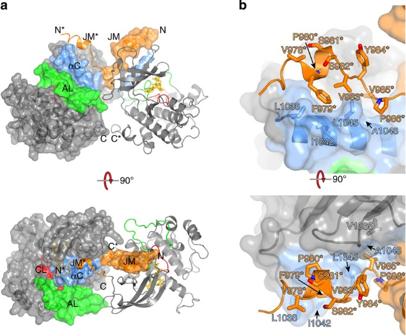Figure 1: Crystal structure of dimeric, autophosphorylated IR-JMTK. (a) Ribbon diagram of a crystallographic dimer of autophosphorylated IR-JMTK. One of the two protomers is shown with a molecular surface. The juxtamembrane region (JM) is coloured orange, the activation loop (AL) is coloured green, the catalytic loop (CL) is coloured red and αC is coloured blue. AMPPCP is coloured yellow and shown in stick representation. An asterisk in the label refers to the second protomer. The N- and C-termini are indicated. The crystallographic two-fold axis is vertical, in the plane of the figure. The view in the lower panel is rotated by 90°, looking from the top. (b) Interactions between the juxtamembrane region of one protomer and the N lobe of the other protomer. Selected residues are shown in stick representation and labelled. The colouring is the same as ina. The view in the upper panel is similar to that in the upper panel ofa, but rotated in the plane of the figure ~45° counterclockwise. The view in the lower panel is rotated by 90° from the upper panel. The protein, to which we added the non-hydrolyzable ATP analogue AMPPCP (Mg 2+ ), crystallized in trigonal space group P3 2 21, with one IR-JMTK molecule in the asymmetric unit ( Table 1 ). Residues 974–1283 could be built into the electron density; residues 956–973 were disordered. The overall structure of the kinase domain is very similar to that in the structure of the phosphorylated IR kinase domain (residues 978–1283) in complex with AMPPNP (Mg 2+ ) and a peptide substrate [12] (PDB code 1IR3); the root-mean-square deviation of Cα atoms is only 0.4 Å. Table 1 X-ray data collection and refinement statistics. Full size table Analysis of the crystal packing of IR-JMTK revealed an interacting molecule, related by a crystallographic two-fold axis ( Fig. 1a ), in which the juxtamembrane region from one molecule binds in the shallow cleft between the β sheet and α-helix C (αC) in the N lobe of the kinase domain from the second molecule, and vice versa ( Fig. 1b and Supplementary Fig. 1a ). This symmetric dimer buries ~2,600 Å of total surface area. Five hydrophobic residues in the juxtamembrane region (Phe979, Pro980, Val983, Val985 and Pro986) interact in trans with four hydrophobic residues in αC (Leu1038, Ile1042, Leu1045 and Ala1048), as well as with Val1065 in β-strand 4 (β4). Intermolecular side-chain interactions between Lys1020 in the β2–3 loop and Asp1156 in the activation loop and between Glu988 and Trp989 at the start of the kinase domain might also contribute to dimer stabilization ( Supplementary Fig. 1b ). Figure 1: Crystal structure of dimeric, autophosphorylated IR-JMTK. ( a ) Ribbon diagram of a crystallographic dimer of autophosphorylated IR-JMTK. One of the two protomers is shown with a molecular surface. The juxtamembrane region (JM) is coloured orange, the activation loop (AL) is coloured green, the catalytic loop (CL) is coloured red and αC is coloured blue. AMPPCP is coloured yellow and shown in stick representation. An asterisk in the label refers to the second protomer. The N- and C-termini are indicated. The crystallographic two-fold axis is vertical, in the plane of the figure. The view in the lower panel is rotated by 90°, looking from the top. ( b ) Interactions between the juxtamembrane region of one protomer and the N lobe of the other protomer. Selected residues are shown in stick representation and labelled. The colouring is the same as in a . The view in the upper panel is similar to that in the upper panel of a , but rotated in the plane of the figure ~45° counterclockwise. The view in the lower panel is rotated by 90° from the upper panel. Full size image Although we have no evidence that phosphorylated IR-JMTK is dimeric in solution, the dimeric architecture of IR and the tethering of the juxtamembrane regions to the transmembrane helices would be conducive to dimerization. Moreover, this dimeric configuration may have functional relevance because αC is an important regulatory element in kinase activation; an intact β3 (lysine)-αC (glutamate) salt bridge is a hallmark of an active protein kinase [16] . Concentration-dependent activation of IR- and IGF1R-JMTK To determine whether the two cytoplasmic domains of IR/IGF1R function as an integrated unit after trans -phosphorylation of the activation loop, we generated constructs encoding hexahistidine-tagged IR-JMTK and IGF1R-JMTK and purified the expressed proteins from baculovirus-infected Spodoptera frugiperda (Sf9) insect cells ( Supplementary Fig. 2a ). For activity assays, we made use of unilamellar vesicles to assemble the JMTK proteins. This experimental system better mimics the quasi-two-dimensional plasma membrane than the cytoplasmic domains in three-dimensional solution (the membrane attachment will significantly enhance the effective concentration for physical interaction), and was used previously to observe the allosteric activation of epidermal growth factor receptor (EGFR) kinase [17] . We first confirmed by native-PAGE that the JMTK proteins were autophosphorylated under the conditions of our assays ( Supplementary Fig. 2b ). Attachment of the purified, autophosphorylated JMTK proteins to the vesicles caused a substantial increase in the activity towards a peptide substrate ( Fig. 2 ). Vesicles that contained no DOGS-NTA-Ni did not produce a significant increase in activity compared with the activity in the absence of vesicles, indicating that the observed effect was not due to an unspecific interaction between the proteins and the lipids. These data show that increasing the local concentration of the proteins increases the catalytic activity towards the substrate, consistent with an activating interaction between two (or more) autophosphorylated JMTK proteins. 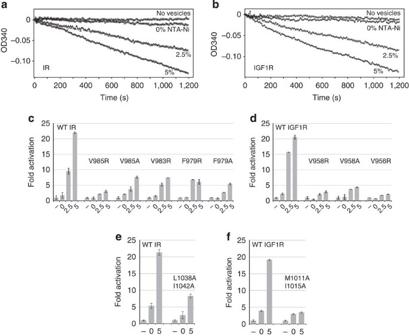Figure 2: Concentration-dependent activation of IR and IGF1R on vesicles. (a) Purified, autophosphorylated His-tagged IR-JMTK was assayed in the presence of lipid vesicles containing the indicated mole ratios of DOGS-NTA-Ni or in the absence of vesicles (−). Enzyme progress curves for phosphorylation of a synthetic peptide substrate were measured using a continuous spectrophotometric assay. The concentrations of enzyme (90 nM) and NTA-Ni (12.5 μM) were kept constant in the assay. (b) Similar experiments were performed for IGF1R-JMTK. (c) Histograms showing rate enhancements for (WT) wild-type and mutant forms of IR-JMTK, relative to control without vesicles. Error bars show s.d. (n=3). (d) Histograms showing rate enhancements for WT and mutant forms of IGF1R-JMTK, relative to the control without vesicles. Error bars show s.d. (n=3). (e) Histograms showing rate enhancements for WT IR-JMTK and a mutant containing amino-acid substitutions in αC in the kinase domain. (f) Same asebut for IGF1R-JMTK. Figure 2: Concentration-dependent activation of IR and IGF1R on vesicles. ( a ) Purified, autophosphorylated His-tagged IR-JMTK was assayed in the presence of lipid vesicles containing the indicated mole ratios of DOGS-NTA-Ni or in the absence of vesicles (−). Enzyme progress curves for phosphorylation of a synthetic peptide substrate were measured using a continuous spectrophotometric assay. The concentrations of enzyme (90 nM) and NTA-Ni (12.5 μM) were kept constant in the assay. ( b ) Similar experiments were performed for IGF1R-JMTK. ( c ) Histograms showing rate enhancements for (WT) wild-type and mutant forms of IR-JMTK, relative to control without vesicles. Error bars show s.d. ( n =3). ( d ) Histograms showing rate enhancements for WT and mutant forms of IGF1R-JMTK, relative to the control without vesicles. Error bars show s.d. ( n =3). ( e ) Histograms showing rate enhancements for WT IR-JMTK and a mutant containing amino-acid substitutions in αC in the kinase domain. ( f ) Same as e but for IGF1R-JMTK. Full size image The crystal structure of IR-JMTK suggests several residues in the juxtamembrane region that should be important for the assembly of the dimer, including Phe979, Val983 and Val985 in IR ( Fig. 1b ) and the equivalent valines, Val956 and Val958, in IGF1R. Using the baculovirus/Sf9 expression system, we produced IR- and IGF1R-JMTK containing amino-acid substitutions at these sites. Autophosphorylation of the mutants occurred with similar kinetics as the wild-type enzymes ( Supplementary Fig. 2b ), indicating that they were not catalytically impaired. After incorporating the mutant proteins into vesicles containing DOGS-NTA-Ni, we measured their catalytic activities towards a peptide substrate. The mutations blunted the increases in enzyme activity that were observed for wild-type IR- and IGF1R-JMTK with increasing mole fraction of DOGS-NTA-Ni ( Fig. 2c,d ), providing evidence that the IR-JMTK crystallographic dimer is relevant in solution. We also mutated residues in αC that, as observed in the crystal structure, interact with the juxtamembrane region to mediate dimer formation (see Fig. 1b ). Leu1038 and Ile1042 in IR (Met1011, Ile1015 in IGF1R) are generally not conserved in RTKs, and these residues were substituted with alanine in the IR-JMTK (L1038A L1042A) and IGF1R-JMTK (M1011A I1015A) proteins. Similar to mutation of residues in the juxtamembrane region, the αC double mutants autophosphorylated normally ( Supplementary Fig. 2b ), but in the vesicle assay, the phosphorylated enzymes were impaired in their ability to phosphorylate a peptide substrate ( Fig. 2e,f ). Single-molecule FRET analysis of IR-JMTK To visualize the interactions between the vesicle-bound, autophosphorylated IR-JMTKs, we performed single-molecule FRET experiments, incorporating the 12-residue sequence for Sfp phosphopantetheinyl transferase [18] at the C-terminus. After expression and purification of modified IR-JMTK from insect cells, we used Sfp to catalyse site-specific transfer of Cy3 or Cy5 dye (from coenzyme A conjugates) onto IR-JMTK ( Supplementary Fig. 2a ). We incubated equal proportions of autophosphorylated IR-JMTK-Cy3 and IR-JMTK-Cy5 with vesicles containing 2.5% DOGS-NTA-Ni and 0.1% biotinylated lipid. The biotinylated vesicles were attached via streptavidin to a passivated microscope slide for imaging. We used excitation at 635 nm to locate vesicles with at least one acceptor Cy5-labelled protein. We then observed these vesicles under 532-nm excitation to identify donor Cy3-labelled proteins and stimulate FRET. All vesicles showing evidence of at least one donor and one acceptor were selected and categorized based on the presence ( Fig. 3a ) or absence of FRET ( Fig. 3b ). We estimated the number of labelled proteins per vesicle by counting steps in the photobleaching decay ( Fig. 3c ). Across all experiments, there was an average of 1.8 labelled proteins per vesicle. Labelling efficiency was typically only 75%, so unlabelled proteins were also present, which would form silent complexes that give no FRET. Because of this uncertainty in stoichiometry for a given vesicle, it was not possible to extract the FRET efficiency or binding rate constants from these measurements. 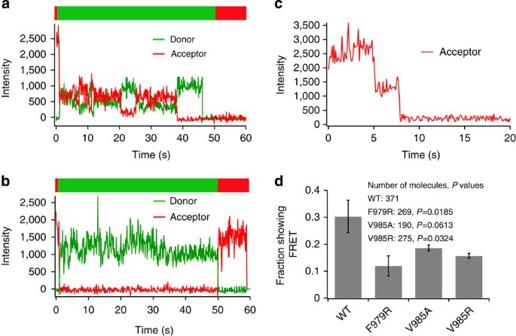Figure 3: Single-molecule FRET analysis of IR-JMTK. Samples traces displaying FRET (a) or no FRET (b) are shown with the laser illumination sequence depicted above the traces. A wavelength of 635 nm (red) is used to locate vesicles with at least one acceptor and 532 nm (green) is used to excite the donor and observe if FRET occurs. A final excitation with 635 nm is used to see if acceptor dyes have been photobleached during donor excitation. (c) Sample trace used for counting steps in the photobleach decay. This vesicle had two labelled acceptors. (d) Fraction of vesicles showing FRET for (WT) wild-type and mutant forms of IR-JMTK. Error bars are±s.d. over three data sets. Figure 3: Single-molecule FRET analysis of IR-JMTK. Samples traces displaying FRET ( a ) or no FRET ( b ) are shown with the laser illumination sequence depicted above the traces. A wavelength of 635 nm (red) is used to locate vesicles with at least one acceptor and 532 nm (green) is used to excite the donor and observe if FRET occurs. A final excitation with 635 nm is used to see if acceptor dyes have been photobleached during donor excitation. ( c ) Sample trace used for counting steps in the photobleach decay. This vesicle had two labelled acceptors. ( d ) Fraction of vesicles showing FRET for (WT) wild-type and mutant forms of IR-JMTK. Error bars are±s.d. over three data sets. Full size image For wild-type protein, ~55% of selected vesicles ( n =3) showed evidence of FRET during 532 nm excitation. Most FRET events were transient, as depicted in Fig. 3a , indicative of reversible binding interactions. Control vesicles lacking DOGS-NTA-Ni showed no evidence of FRET. We carried out similar experiments on Cy3- and Cy5-labelled mutant forms of IR-JMTK. These mutations (F979R, V985A/R) are in the interface of the IR-JMTK crystallographic dimer ( Fig. 1b ). Consistent with the decrease in concentration-dependent activation ( Fig. 2c,d ), the point mutations also reduced the frequency of FRET events by 50% or more relative to the wild-type protein ( Fig. 3d ). Optimal IRS-1 phosphorylation depends on IR-JMTK dimer Finally, we tested the importance of the activated JMTK dimer for substrate phosphorylation in the context of full-length IR expressed in mammalian cells. Expression of wild-type IR in HEK293T cells and stimulation with insulin led to receptor autophosphorylation and tyrosine phosphorylation of a 180-kDa protein ( Fig. 4a ), which we confirmed was IRS-1 ( Supplementary Fig. 2c ). Autophosphorylation of the kinase dimer-disrupting F979A/R, V983R and V985R mutant forms of IR was stimulated by insulin similar to wild-type IR ( Fig. 4b ), but phosphorylation of IRS-1 by these mutants was markedly diminished ( Fig. 4a,c ). This defect in protein–substrate phosphorylation is consistent with the results of the in vitro vesicle experiments ( Fig. 2c,d ), in which the mutations interfered with the concentration-dependent increase in peptide-substrate phosphorylation. 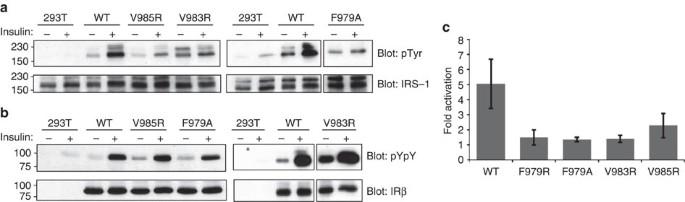Figure 4: Dimerization of IR-JMTK potentiates IRS-1 phosphorylation. HEK293T cells expressing wild-type (WT) or mutant forms of full-length IR were starved overnight, then stimulated with insulin or left untreated. Cell lysates were analysed by western blotting with the indicated antibodies (pTyr, 4G10; pYpY, pTyr1162–1163). (a) IRS-1 tyrosine phosphorylation. (b) IR autophosphorylation. The results shown are representative of four independent experiments (the samples used in the blots inaare the same as those used in the blots inb). The positions of molecular weight markers (in kDa) are indicated on the left-sides of the blots. (c) Quantification of insulin-stimulated IRS-1 phosphorylation. Error bars show s.d. (n=3). Figure 4: Dimerization of IR-JMTK potentiates IRS-1 phosphorylation. HEK293T cells expressing wild-type (WT) or mutant forms of full-length IR were starved overnight, then stimulated with insulin or left untreated. Cell lysates were analysed by western blotting with the indicated antibodies (pTyr, 4G10; pYpY, pTyr1162–1163). ( a ) IRS-1 tyrosine phosphorylation. ( b ) IR autophosphorylation. The results shown are representative of four independent experiments (the samples used in the blots in a are the same as those used in the blots in b ). The positions of molecular weight markers (in kDa) are indicated on the left-sides of the blots. ( c ) Quantification of insulin-stimulated IRS-1 phosphorylation. Error bars show s.d. ( n =3). Full size image Although a structural characterization of the IR/IGF1R signal-transduction mechanism is still lacking, it is well established that insulin/IGF1 binding to the ectodomain of its receptor induces tyrosine phosphorylation of the activation loop (and juxtamembrane region) in the cytoplasmic tyrosine kinase domains, which stimulates catalytic activity [4] . Whether the phosphorylated kinase domains then function independently or cooperatively to phosphorylate downstream substrates such as IRS-1 was not known. Previously reported crystal structures of the phosphorylated kinase domains of IR (PDB code 1IR3 (ref. 12 )) and IGF1R (PDB code 1K3A [13] ) contain one molecule in the asymmetric unit and do not contain packing configurations that are suggestive of possible activated dimers. Here we describe a crystal structure of the IR kinase domain with an intact juxtamembrane region, in which a possible activated dimer presents itself in the crystal. In this symmetric dimer, the juxtamembrane region of one protomer interacts with the N lobe of the other protomer ( Fig. 1 ). Of note, the phosphorylated IR kinase domain crystallized in a very similar lattice (PDB code 1IR3 (ref. 12 )) and contains the same crystallographic dimer, but because of the shorter juxtamembrane segment (starting residue 978 instead of 956), the buried surface area is less (1,770 Å 2 versus 2,600 Å 2 ). The crystal structure of phosphorylated IGF1R kinase (PDB code 1K3A [13] ), which lacks in the construct the majority of the juxtamembrane region, does not show this dimeric configuration. On the basis of the previous structures of the unphosphorylated IR and IGF1R kinase domains and the current structure of phosphorylated IR-JMTK, we propose that the juxtamembrane region of IR and IGF1R functions as both a cis -autoinhibitory element and a trans -activation element ( Fig. 5a,b ). As described previously [14] , in the unphosphorylated (basal) state of the IR kinase, the juxtamembrane region interacts (in cis ) with αC, anchored by Tyr984 (not an autophosphorylation site) in the juxtamembrane segment proximal to the kinase domain ( Fig. 5a ). Mutation of Tyr984 (or Tyr957 in IGF1R) results in a substantial increase in catalytic activity [14] , [15] , in part, because Tyr984 stabilizes a non-productive position of αC, in which the β3-αC (Lys1030-Glu1047 in IR) salt bridge is not formed ( Fig. 5a ). Whether in the basal state the kinase domains are spatially separated (monomeric) or form an inhibitory dimer is not known. 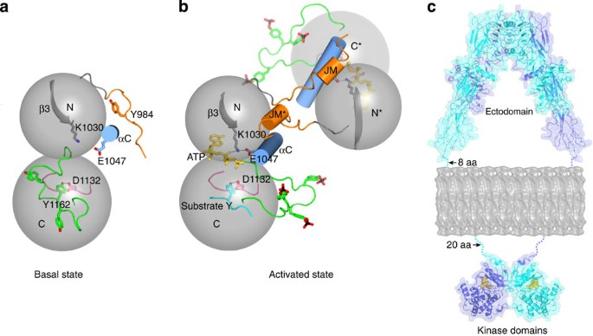Figure 5: Model for IR/IGF1R juxtamembranecis-autoinhibition andtrans-activation. (a) In the basal (unphosphorylated) state of the kinase domain, the activation loop (green) is autoinhibitory, binding as a substrate (Tyr1162) in its own active site (Asp1132 in the catalytic loop (pink)) in the C lobe (‘C’). Tyr984 in the juxtamembrane region (orange) binds in the cleft between the β sheet and αC (blue) in the kinase N lobe (‘N’), stabilizing an αC position that is unfavourable for the formation of the β3 (Lys1030)-αC (Glu1047) salt bridge. Only one kinase domain of the dimeric receptor is shown. (b) On insulin/IGF1-inducedtrans-phosphorylation of the activation loop and reconfiguration, the juxtamembrane region crosses over to bind in the β sheet-αC cleft of the neighbouring kinase domain, stabilizing a position of αC that promotes the formation of the Lys1030-Glu1047 salt bridge, which in turn facilitates binding of Lys1030 to phosphates of ATP (yellow) and substrate (cyan) phosphorylation. An asterisk in the label refers to the second protomer. (c) Structural model of activated IR. The IR ectodomain structure is of the basal, apo form (the only full-length IR ectodomain structure available; PDB code 3LOH (ref.26)). One half-receptor (consisting of both α and β subunits) is coloured cyan and the other half-receptor is coloured purple. Eight amino acids (depicted by a dashed line) connect the ends of the third fibronectin type III domains to the transmembrane helices (not shown). A membrane bilayer is depicted (to scale) in grey. The protomers of the IR-JMTK dimer are coloured cyan and purple, and AMPPCP (marking the active sites) is shown in sphere representation and coloured yellow. Twenty amino acids (depicted by a dashed line) connect the transmembrane helices to the juxtamembrane region at the start of the JMTK crystal structure. Figure 5: Model for IR/IGF1R juxtamembrane cis -autoinhibition and trans -activation. ( a ) In the basal (unphosphorylated) state of the kinase domain, the activation loop (green) is autoinhibitory, binding as a substrate (Tyr1162) in its own active site (Asp1132 in the catalytic loop (pink)) in the C lobe (‘C’). Tyr984 in the juxtamembrane region (orange) binds in the cleft between the β sheet and αC (blue) in the kinase N lobe (‘N’), stabilizing an αC position that is unfavourable for the formation of the β3 (Lys1030)-αC (Glu1047) salt bridge. Only one kinase domain of the dimeric receptor is shown. ( b ) On insulin/IGF1-induced trans -phosphorylation of the activation loop and reconfiguration, the juxtamembrane region crosses over to bind in the β sheet-αC cleft of the neighbouring kinase domain, stabilizing a position of αC that promotes the formation of the Lys1030-Glu1047 salt bridge, which in turn facilitates binding of Lys1030 to phosphates of ATP (yellow) and substrate (cyan) phosphorylation. An asterisk in the label refers to the second protomer. ( c ) Structural model of activated IR. The IR ectodomain structure is of the basal, apo form (the only full-length IR ectodomain structure available; PDB code 3LOH (ref. 26 )). One half-receptor (consisting of both α and β subunits) is coloured cyan and the other half-receptor is coloured purple. Eight amino acids (depicted by a dashed line) connect the ends of the third fibronectin type III domains to the transmembrane helices (not shown). A membrane bilayer is depicted (to scale) in grey. The protomers of the IR-JMTK dimer are coloured cyan and purple, and AMPPCP (marking the active sites) is shown in sphere representation and coloured yellow. Twenty amino acids (depicted by a dashed line) connect the transmembrane helices to the juxtamembrane region at the start of the JMTK crystal structure. Full size image Among other effects, phosphorylation of the activation loop (and the conformational changes that result) promotes the pivoting of αC towards the active site, which facilitates the formation of the β3-αC salt bridge ( Fig. 5b ). Concomitantly, the interaction between the juxtamembrane region and αC (of the same molecule) is destabilized. We hypothesize that this facilitates ‘cross-over’ of the juxtamembrane region to the N lobe of the other kinase domain (the specific cis and trans interactions between the juxtamembrane region and αC are distinct), which stabilizes the β3-αC salt bridge ( Fig. 5b ) and accounts for the higher activity of the kinase domain towards substrates ( Figs 2 and 4 ). Indeed, in the IGF1R activation study [9] , k cat for substrate-peptide phosphorylation was four-fold higher for a juxtamembrane-kinase domain construct than for the kinase domain alone. Thus, kinase activation in IR and IGF1R involves both activation-loop phosphorylation and allosteric stabilization through dimer formation. Consistent with a putative activated dimer, the two N-termini (Ser974) point in the same direction (towards the membrane; 41 Å apart) and the two active sites are accessible to substrates ( Fig. 5c ). Because 20 residues of unknown structure link the transmembrane helices to the crystallographic JMTK dimer, this dimer is compatible with (or cannot distinguish between) either of the two insulin-induced receptor-activation mechanisms mentioned previously: transmembrane-helix separation [8] or dimerization [9] . Interestingly, the juxtamembrane region of IR from mammalian species contains a five-residue insertion relative to IR from other species and relative to IGF1R ( Supplementary Fig. 3 ; the juxtamembrane region is otherwise well conserved between IR and IGF1R), the residues of which (978–982) form the short α helix that binds to αC (in trans ; Fig. 1b ). IR-related receptor is also missing these five residues, as are the single insulin/IGF1 receptors in invertebrates. The absence of these five residues in the juxtamembrane region of IGF1R (and of the other receptors) probably alters the precise mode of interaction between the juxtamembrane region and the kinase domain to mediate dimer formation, but the mutational data for IGF1R ( Fig. 2 ) indicate a similar allosteric outcome. Furthermore, the invertebrate receptors lack one or more of the hydrophobic residues in the juxtamembrane region or αC ( Supplementary Fig. 3 ), suggesting that allosteric stabilization of the kinase domains is a feature of vertebrate IR/IGF1R. For many other RTKs, such as fibroblast growth factor receptors, TrkA-C and MuSK, activation-loop phosphorylation is an essential aspect of kinase activation. Whether kinase dimerization also contributes to the activation of these RTKs is not known. If so, the dimerization mode is probably different than that for IR/IGF1R, given that there is no obvious sequence conservation between the juxtamembrane region of IR/IGF1R and of these other RTKs, and two of the hydrophobic residues in αC (Leu1038 and Ile1042) that mediate IR kinase dimerization ( Fig. 1b ) are also not conserved. The kinase activation mechanism for IR and IGF1R is distinct from that for EGFR, in which activation-loop phosphorylation plays at most a minor role, and the predominant activation mechanism is ligand-induced formation of an asymmetric kinase dimer prior to autophosphorylation (of the carboxy (C)-terminal tail of the receptor) [19] . One aspect in common between the two mechanisms is the involvement of αC, which in EGFR is stabilized in the active position by the C lobe of the second kinase domain and in IR/IGF1R by the juxtamembrane region of the other β subunit ( Supplementary Fig. 4 ). The discovery reported here on the dimeric, active form of the IR kinase raises the possibility of identifying small molecules that could bind in the β sheet-αC cleft of the kinase N lobe, simultaneously displacing autoinhibitory Tyr984 and stabilizing the β3-αC salt bridge. Such compounds could serve as cytoplasmic activators of IR and potentially find use as novel therapeutics in the treatment of type 2 diabetes mellitus. Expression and purification of IR- and IGF1R-JMTK For structural studies, residues 956–1283 of human IR, which includes the full juxtamembrane region (residues 956–989) and the tyrosine kinase domain (residues 989–1283), were cloned into a pFastBac vector (Life Technologies). Two mutations were introduced, C981S and Y965F, to avoid artifactual disulfide-bond formation and heterogeneous tyrosine phosphorylation, respectively. Mutagenesis was performed using QuikChange site-directed mutagenesis kit (Stratagene) and verified by DNA sequencing. A recombinant baculovirus expressing IR-JMTK was constructed using the Bac-to-Bac system (Life Technologies). IR-JMTK was purified from baculovirus-infected Sf9 insect cells as described previously in ref. 10 . In vitro phosphorylation of IR-JMTK was performed by incubating the protein with 10 mM ATP and 25 mM MgCl 2 , and the reaction was followed by native-PAGE. Tetra-phosphorylated IR-JMTK (pTyr972, pTyr1158, pTyr1162 and pTyr1163) was purified using Mono-Q anion-exchange chromatography (GE Healthcare). The phosphorylation state of IR-JMTK was verified by mass spectrometry. For in vitro assays, DNAs encoding residues 930–1256 of human IGF1R and 953–1283 of human IR were cloned into pFastBac HTb (Life Technologies) using the BamHI and HindIII restriction sites. The resulting constructs contain an amino (N)-terminal His 6 tag. All mutations were introduced using QuikChange according to the manufacturer’s protocols. Sequences of all the plasmids were verified by DNA sequencing, after which the recombinant viruses were generated using the Bac-to-Bac system (Life Technologies). Sf9 cells were infected with recombinant baculovirus and collected after 72 h of infection. The proteins were purified as described previously in ref. 15 . Crystallization and X-ray data collection Crystals of IR-JMTK were obtained by hanging-drop vapour diffusion at 4 °C by mixing 2 μl of tetra-phosphorylated IR-JMTK (4 mg ml −1 ), containing 2 mM AMPPCP and 6 mM MgCl 2 , with 1 μl of reservoir solution (100 mM Tris-HCl, pH 7.5, 26% (w/v) polyethylene glycol 4000, 200 mM MgCl 2 and 5 mM DTT). The crystals belong to trigonal space group P3 2 21 ( Table 1 ) with one IR-JMTK molecule per asymmetric unit (solvent content of 48%). IR-JMTK crystals were soaked in a series of cryoprotectant solutions with increasing ethylene glycol concentration (5, 10 and 15%) before being flash-frozen in a dry nitrogen stream at 100 K. X-ray diffraction data were collected at beam line X12C at the National Synchrotron Light Source, Brookhaven National laboratory. The structure was solved by molecular replacement using AMoRe [20] , with phosphorylated IR kinase (PDB code I1R3 (ref. 12 )) used as a search model. Iterative rounds of model building in Coot [21] and positional and B-factor refinement with REFMAC [22] led to an atomic model of IR-JMTK at 2.3-Å resolution consisting of IR residues 974–1283 (956–973 are disordered), one AMPPCP molecule, two Mg 2+ ions and 141 water molecules. Preparation of unilamellar vesicles Egg phosphatidylcholine and DOGS-NTA-Ni (Avanti Polar Lipids) were mixed in different molar ratios (0, 2.5 and 5%) in a glass tube. A thin lipid film was formed on evaporating chloroform under an argon gas stream and the lipids were dried under vacuum overnight. The dried lipids were resuspended by adding 220 μl of rehydration buffer (20 mM Tris-HCl, pH 7.5 and 150 mM NaCl) followed by at least five freeze–thaw cycles and 30 s vigorous vortexing to convert the lipid film into large, multilamellar vesicles. After incubation for 3 h in rehydration buffer, homogeneous small unilamellar vesicles were formed by passing the large multilamellar vesicles through a polycarbonate filter (pore size: 100 nm) 21–41 times, using a mini-extruder (Avanti Polar Lipids). The vesicles were used for in vitro assays on the same day of preparation. In vitro kinase assays A continuous enzyme-coupled kinase assay was performed to measure the kinase activity of the proteins as described in refs 23 , 24 , with minor modifications. Reactions were carried out at 30 °C in a final volume of 50 μl containing 100 mM Tris-HCl, pH 7.4, 10 mM MgCl 2 , 2 mM ATP, 1.5 mM phosphoenolpyruvate, 90 units per ml pyruvate kinase, 109 units per ml lactate dehydrogenase, 1.2 mg ml −1 NADH and 90 nM IR- or IGF1R-JMTK. For all assays with DOGS-NTA-Ni containing vesicles, the total concentration of the DOGS-NTA-Ni in the bulk solution was kept at 12.5 μM. Proteins and vesicles were preincubated at 4 °C for 15 min, then the complexes were autophosphorylated at room temperature by incubation with 1 mM ATP in 20 mM Tris-HCl, pH 7.5 and 10 mM MgCl 2 before starting the kinase assay. Reactions were initiated by the addition of 55 μM peptide substrate (KKEEEEYMMMM). Preparation of fluorescently labelled IR-JMTK Cy3 or Cy5 dyes were incubated with coenzyme A (1.5-fold molar excess) for 3 h in 100 mM sodium phosphate, pH 7.0. The fluorophore-CoA conjugates were purified by semi-preparative high-performance liquid chromatography on a C18 column. The recognition sequence for Sfp transferase (GDSLSWLLRLLN) [25] was inserted at the C-terminus of IR-JMTK by site-directed mutagenesis, and the modified protein was expressed and purified from Sf9 cells as described above. Sfp was expressed and purified from Escherichia coli as described in ref. 18 . For protein labelling, Sfp (1 μM) was incubated with 45 μM IR-JMTK and 45 μM fluorophore-CoA conjugate for 30 min at room temperature in a buffer containing 20 mM Tris-HCl, pH 7.5, 10 mM MgCl 2 and 150 mM NaCl. The labelled protein was purified on a Sephadex-G25 column. To detect fluorophore labelling, fractions were analysed by 10% SDS–PAGE and detected by imaging (FluorChem E Imager, ProteinSimple) and Coomassie blue staining. The spectrum of each fraction was measured in a ultraviolet/visible spectrophotometer and the degree of labelling was calculated using the extinction coefficient of each fluorophore and the absorbance at 554 and 649 nm for Cy3 and Cy5, respectively. Single-molecule FRET measurements of IR-JMTK IR-JMTK-Cy3 (80 μg ml −1 ) and IR-JMTK-Cy5 (80 μg ml −1 ) were incubated with vesicles containing 2.5% DOGS-NTA-Ni and 0.1% biotin phosphatidylethanolamine (16 μg ml −1 ) at 4 °C for 15 min. IR-JMTK-Cy3/5 was autophosphorylated by incubation with 20 mM Tris-HCl, pH 7.5, 100 μM ATP, 5 mM MgCl 2 and 150 mM NaCl for 5 min at room temperature. The vesicles were purified on a C4LB column, then immobilized by a biotin-streptavidin linkage on quartz slides that had been passivated with biotinylated bovine serum albumin to prevent non-specific binding. Samples were diluted to picomolar concentrations to achieve optically resolved vesicles. Images were collected using a 60X, 1.2 NA water immersion objective (Olympus), and recorded with an Andor iXon EMCCD camera (Andor Technologies) at a frame rate of 10 Hz. Vesicles were imaged in 20 mM Tris-HCl, pH 7.5 and 150 mM NaCl supplemented with 0.1% glucose, 5 mM cyclooctatetraene (a triplet state quencher), 0.2 units per μl glucose oxidase and 2 units per μl catalase as an oxygen scavenging system to delay photobleaching. Excitation at 635 nm was used to locate acceptor dyes followed by excitation with 532 nm at ~7 mW to record FRET. Vesicles displaying evidence of at least one donor and one acceptor were selected and categorized by the presence or absence of FRET during donor excitation. For each data set, fraction showing FRET was normalized by setting the wild type to one. Number of donors/acceptors per vesicle was determined by counting steps in the photobleach decay. All samples had an average of 1–2 donors and acceptors per vesicle. IRS-1 phosphorylation in mammalian cells Human embryonic kidney 293T cells were cultured in Dulbecco's modified Eagle's medium supplemented with 10% fetal bovine serum. The full-length human IR cDNA (exon 11- form) was cloned into plasmid pCMV-HA (Clontech). Site-directed mutations were introduced using QuikChange. Cells were transfected with the appropriate plasmids using X-treme GENE HP DNA transfection reagent (Roche), according to the manufacturer's instructions. Whole-cell lysates were prepared using a buffer containing 1% NP40, 25 mM Tris-HCl, pH 7.5, 100 mM NaCl and 1 mM EDTA. The following antibodies were used for western blotting: anti-phosphotyrosine, clone 4G10 (cat. no. 05-321, Millipore) at 1:2,000 dilution, anti-IRβ, C-19 (cat. no. sc-711, Santa Cruz Biotechnology) at 1:1,000 dilution, anti-IRS-1 (cat. no. 07-843, Millipore) at a concentration of 0.75 μg ml −1 and anti-phospho-IR (pTyr1162/pTyr1163; cat. no. 44804G, Life Technologies) at 1:5,000 dilution. Subsequently, membranes were washed and incubated with horseradish peroxidase-conjugated secondary antibody. After washing several times, the membranes were developed with an enhanced chemiluminescence (ECL) system according to the manufacturer's instructions (Thermo Scientific). Accession codes : Atomic coordinates and structure factors for the IR-JMTK structure have been deposited in the Protein Data Bank with ID code 4XLV . How to cite this article: Cabail, M. Z. et al . The insulin and IGF1 receptor kinase domains are functional dimers in the activated state. Nat. Commun . 6:6406 doi: 10.1038/ncomms7406 (2015).